RETRACTED ARTICLE: Polymerase θ inhibition activates the cGAS-STING pathway and cooperates with immune checkpoint blockade in models of BRCA-deficient cancer Recently developed inhibitors of polymerase theta (POLθ) have demonstrated synthetic lethality in BRCA-deficient tumor models. To examine the contribution of the immune microenvironment to antitumor efficacy, we characterized the effects of POLθ inhibition in immunocompetent models of BRCA1-deficient triple-negative breast cancer (TNBC) or BRCA2-deficient pancreatic ductal adenocarcinoma (PDAC). We demonstrate that genetic POLQ depletion or pharmacological POLθ inhibition induces both innate and adaptive immune responses in these models. POLθ inhibition resulted in increased micronuclei, cGAS/STING pathway activation, type I interferon gene expression, CD8 + T cell infiltration and activation, local paracrine activation of dendritic cells and upregulation of PD-L1 expression. Depletion of CD8 + T cells compromised the efficacy of POLθ inhibition, whereas antitumor effects were augmented in combination with anti-PD-1 immunotherapy. Collectively, our findings demonstrate that POLθ inhibition induces immune responses in a cGAS/STING-dependent manner and provide a rationale for combining POLθ inhibition with immune checkpoint blockade for the treatment of HR-deficient cancers. Tumors deficient in homologous recombination (HR) repair secondary to mutations in genes such as BRCA1 or BRCA2 , are dependent on alternative DNA damage response (DDR) pathways to maintain genomic integrity, rendering them susceptible to synthetic lethal targeting of these pathways [1] , [2] , [3] . Over the past several years, the principle of synthetic lethality has been successfully employed as a therapeutic strategy, leading to the FDA approval of inhibitors of poly (ADP-ribose) polymerase (PARP) for clinical use in BRCA-deficient breast, ovarian, pancreatic, and prostate cancers [4] . More recently, inhibitors of polymerase theta (POLθ, encoded by POLQ ), the critical enzyme in microhomology-mediated end-joining (MMEJ), have been shown to abrogate MMEJ, and are similarly synthetic lethal in tumors with HR repair deficiency [5] , [6] . The dependence of HR repair-deficient cancers on MMEJ is reflected by their high levels of POLθ expression [7] , [8] . Furthermore, HR-deficient tumors that acquire resistance to PARP inhibition may retain increased POLθ expression and MMEJ dependence, so that POLθ inhibition may overcome PARP inhibitor resistance [5] . Multiple cell-intrinsic and cell-extrinsic mechanisms account for the synthetic lethality between PARP inhibition or POLθ inhibition and HR-deficiency [4] , [9] , [10] , [11] . Regarding cell-extrinsic mechanisms, DNA damage mediated by PARP inhibition in BRCA1-deficient cancers induces T-cell infiltration and activation via the cyclic GMP-AMP synthase (cGAS)/stimulator of interferon genes (STING) innate immunity pathway, leading to increased expression of type I interferons [12] , [13] . Consequently, the addition of PD-1 or PD-L1 blockade enhances the therapeutic efficacy of PARP inhibition in preclinical models [12] , [13] , [14] , [15] . Notably, Polq knockout mice exhibit increased micronucleation [16] , [17] and therefore a source of immunostimulatory DNA. Based on this phenotype, as well as the synthetic lethality between POLθ inhibition and HR-deficiency, and recent data demonstrating activation of the cGAS/STING pathway upon combined knockout of POLQ and FANCD2 in esophageal cancers [18] , we hypothesized that POLθ inhibition in BRCA-deficient cancers would likewise activate the cGAS/STING pathway and lead to increased T-cell infiltration and activation, with sensitization to immune checkpoint blockade. In this study, we used human cell lines and mouse models representative of BRCA1-deficient triple-negative breast cancer (TNBC) and BRCA2-deficient pancreatic ductal adenocarcinoma (PDAC) to demonstrate that pharmacological inhibition of POLθ using either novobiocin (NVB), an inhibitor of the POLθ ATPase domain for which we have previously established biochemical and biological specificity [5] , or ART558, an inhibitor of the POLθ polymerase domain [6] , as well as genetic depletion of POLQ , all induce cGAS/STING pathway activation. Consequently, POLθ inhibition drives the expression of type I interferon response elements, including PD-L1, and increases CD8 + T-cell tumor infiltration and activation, as well as activation of antigen-presenting dendritic cells (DCs) in a paracrine fashion. Depletion of CD8 + T cells decreased the antitumor efficacy of NVB. In contrast, the antitumor activity of NVB was augmented with the addition of an anti-PD-1 antibody. Thus, our study uncovers a novel mechanism contributing to the activity of POLθ inhibition in BRCA-deficient breast and pancreatic cancers that is mediated by host immune responses and that can be enhanced by immune checkpoint blockade. POLθ inhibition enhances PD-L1 expression in vitro and in vivo and synergizes with anti-PD-1 immunotherapy in HR-deficient cancers Given the synthetic lethal relationship between HR deficiency and POLθ inhibition, as well as the known stimulation of antitumor immune responses by DNA damage, we hypothesized that POLθ inhibition would promote antitumor immunity [7] , [19] , [20] . To investigate the interactions of POLθ inhibition with the immune microenvironment in HR-deficient cancers, we first determined the effect of POLθ inhibition on PD-L1 expression in two different BRCA-deficient cancer cell lines. We treated both BRCA1-deficient MDA-MB-436 TNBC cells and BRCA2-deficient CAPAN-1 PDAC cells with the POLθ ATPase domain inhibitor NVB and analyzed PD-L1 expression by immunoblot and quantitative PCR (qPCR) [5] . Treatment with NVB significantly increased the total level of PD-L1 protein (Fig. 1a, b , left panels) and CD274/PDL1 mRNA expression (Fig. 1a, b , right panels) in both cell lines. To confirm that PD-L1 induction was specifically due to POLθ inhibition by NVB and not by an off-target effect, we also knocked down POLQ using siRNA in both MDA-MB-436 and CAPAN-1 cells. Consistent with NVB-mediated pharmacological inhibition, PD-L1 expression was increased in POLQ- depleted MDA-MB-436 (Supplementary Fig. 1a ) and CAPAN-1 (Supplementary Fig. 1b ) cells. In addition, PD-L1 upregulation upon POLθ inhibition was confirmed by treatment of MDA-MB-436 (Supplementary Fig. 1c ) and CAPAN-1 cells (Supplementary Fig. 1d ) with an inhibitor of the POLθ polymerase domain, ART558, demonstrating that results are similar regardless of the use of an ATPase inhibitor or a polymerase domain inhibitor of POLθ [6] . Fig. 1: POLθ inhibition induces PD-L1 expression in vitro and in vivo and is enhanced by anti-PD-1 immunotherapy in HR-deficient cancers. a – d BRCA1- mutant MDA-MB-436 TNBC ( a ) cells, or BRCA2- mutant CAPAN-1 PDAC ( b ) cells, and their isogenic pairs, BRCA1-expressing MDA-MB-436 ( c ), or BRCA2-expressing CAPAN-1 ( d ), were exposed to 100 μM novobiocin (NVB) for 48 h. Left: Immunoblot for PD-L1 expression. Right: Quantification of PD-L1 mRNA levels by RT-qPCR. Transcript levels are measured relative to ACTB by qPCR. Data, mean +/− SD of three independent experiments, unpaired two-tailed t- test. e Tumor chunks derived from the K14-Cre-Brca1 f/f ;Trp53 f/f GEMM were transplanted in syngeneic FVB/129P2 mice treated with vehicle (VEH, n = 5) or NVB ( n = 7) at 75 mg/kg via intraperitoneal (IP) injection twice daily, were harvested after 5 days of treatment for PD-L1 expression by IHC. Staining was quantified using Aperio algorithms. (Left: Representative IHC images at 40x magnification, scale bars, 100 μM. Right: Quantification, Data, mean +/− SEM, unpaired two-tailed t- test. f Immunoblot analysis of Brca2 protein expression in CRISPR knockout Kras LSL-G12D ; TP53 LoxP ; Pdx1-Cre; Rosa26YFP/YFP (KPC) cells. Vinculin serves as an internal loading control. Representative immunoblot of three independent experiments. g Brca2 KO KPC cells were injected into the flanks of syngeneic C57BL/6 mice and treated with VEH( n = 5) or NVB ( n = 5) at 75 mg/kg via IP injection twice daily. After 5 days of treatment, tumors were harvested and subjected to IHC for PD-L1 expression. Left: Representative IHC images at 40x magnification, scale bars, 100 μM. Right: Quantification, Data, mean +/− SEM, unpaired two-tailed t- test. h , i PD-L1 protein ( h ) or mRNA ( i ) expression in K14-Cre-Brca1 f/f ;Trp53 f/f TNBC tumors. VEH, n = 7; NVB, n = 6 in ( h ); VEH, n = 9; NVB, n = 9 in ( i ). j , k PD-L1 protein ( j ) or mRNA ( k ) expression in Brca2 KO KPC PDAC tumors. VEH, n = 10; NVB, n = 9 in ( j ); VEH, n = 5; NVB, n = 5 in k . Error bars, SEM. Statistical analyses were performed using unpaired two-tailed t -tests. l Brca2 KO KPC tumor-bearing syngeneic C57BL/6 mice were treated with VEH ( n = 11) or NVB (75 mg/kg IP twice daily, n = 10), along with isotype control ( n = 11) or an anti-PD-1 antibody (200 µg twice weekly, n = 11) for 28 days, and serial fold-change in tumor volume was recorded. Data, mean +/− SEM, one-way ANOVA analysis. m Kaplan–Meier analysis for time until tumor progression necessitated euthanasia. Median survivals are shown in parentheses for mice from 1l . Kaplan–Meier curves were analyzed by the log-rank test. Full size image We next determined whether upregulation of PD-L1 upon NVB treatment requires the synthetic lethal relationship between HR-deficiency and POLθ inhibition. We reasoned that upregulation of PD-L1 expression would be abrogated if this relationship were rescued by HR proficiency. To investigate this hypothesis, we utilized isogenic pairs of parental and BRCA1 or BRCA2-reconstituted MDA-MB-436 and CAPAN-1 cells [21] , [22] . Treatment with NVB did not increase the total level of PD-L1 protein in BRCA1-reconstituted MDA-MB-436 cells or BRCA2-reconstituted CAPAN-1 cells by immunoblot analysis (Fig. 1c, d , left panels). These results were again validated by quantitative PCR, demonstrating absence of increased CD274/PDL1 expression with NVB treatment in BRCA-reconstituted cells (Fig. 1c, d , right panels). The underlying mechanism of this loss of increased PD-L1 expression is likely decreased POLQ expression in BRCA-reconstituted (i.e., HR-proficient) cancer cells (Supplementary Fig. 1e, f ), which correlates with decreased sensitivity to NVB-mediated POLθ inhibition [7] , [8] . To determine whether NVB-mediated POLθ inhibition in HR-deficient cancer cells would upregulate PD-L1 expression in vivo, we employed two HR-deficient immunocompetent mouse models. To recapitulate BRCA1 deficiency in breast cancer, tumors derived from the K14-Cre-Brca1 f/f ; Trp53 f/f immunocompetent genetically engineered mouse model of TNBC were orthotopically implanted into the mammary fat pads of FVB/129P2 syngeneic mice. To recapitulate BRCA2 deficiency in pancreatic cancer, Brca2 was knocked out by CRISPR/Cas9 in a murine PDAC cell line derived from late-stage primary tumors from an autochthonous mouse model of Kras G12D and Trp53 R172H -mutated PDAC (KPC) [23] (Fig. 1f ). Brca2 -null KPC cells were subcutaneously injected into immunocompetent C57BL/6 mice. In both models, mice were treated with vehicle or NVB for 5 days. Analysis of Brca1-deficient breast tumors from NVB-treated mice demonstrated significant upregulation of PD-L1 expression by immunohistochemistry (IHC) (Fig. 1e ) and by flow cytometry (Fig. 1h ; Supplementary Fig. 1g, h ). Whole-tumor Cd274/Pd-l1 mRNA expression was also significantly increased in NVB-treated mice compared to vehicle-treated mice (Fig. 1i ). Consistent with these results, Brca2-deficient PDAC from NVB-treated mice also demonstrated significantly upregulated PD-L1 expression by IHC (Fig. 1g ) and by flow cytometry (Fig. 1j ). Similarly, whole-tumor Cd274/Pdl1 mRNA expression was significantly increased in NVB-treated compared to vehicle-treated mice (Fig. 1k ). Altogether, these results demonstrate that NVB-mediated POLθ inhibition upregulates PD-L1 expression in HR-deficient cancers both in vitro and in vivo. Given that PD-L1 expression was significantly increased following NVB treatment in HR-deficient cancers both in vitro and in vivo, we hypothesized that PD-1 blockade might augment the antitumor activity of NVB. Brca2-deficient KPC cells were subcutaneously injected into immunocompetent C57BL/6 and treated with vehicle or NVB, with or without anti-PD-1 blockade, for 28 days, all of which were well tolerated (Supplementary Fig. 1i ). Mice treated with vehicle or anti-PD-1 alone showed no antitumor response. Mice treated with NVB-alone demonstrated tumor growth inhibition (Fig. 1l ) and overall survival (Fig. 1m ) that was significantly improved with the addition of anti-PD-1 blockade. Thus, NVB-mediated POLθ inhibition increases PD-L1 expression and demonstrates enhanced antitumor activity when combined with anti-PD-1 immunotherapy in HR-deficient cancers. Efficacy of POLθ inhibition in HR-deficient cancers requires CD8 + T cells Given the effects of NVB-mediated POLθ inhibition on PD-L1 expression and the interaction with anti-PD-1 blockade in HR repair-deficient cancers, we reasoned that the antitumor activity of NVB may depend on tumor cell-extrinsic responses in addition to the known cell-intrinsic mechanisms. To this end, we sought to further characterize the effects of NVB on the tumor immune microenvironment of Brca1-deficient TNBC and Brca2-deficient PDAC by IHC and flow cytometry, with particular emphasis on T-cell subsets given the induction of PD-L1 upon POLθ inhibition (Fig. 1 ). IHC analyses of Brca1-deficient TNBC or Brca2-deficient PDAC tumors from NVB-treated immunocompetent mice showed increased CD3 + , CD4 + , and CD8 + T-cell infiltrates (Fig. 2a, b ), confirmed in both models by flow cytometry (Fig. 2c–f ; Supplementary Fig. 2a–d ). Importantly, the recruited CD8 + T cells were cytolytically active, as demonstrated by increased Granzyme B staining (Fig. 2c, d ). Although the number of CD4 + T cells was increased, the proportion of regulatory FOXP3 + , CD4 + T cells (Treg) was not significantly affected, suggesting that conventional CD4 + T were recruited and may also contribute to NVB-mediated antitumor effects (Fig. 2e, f ). Indeed, many types of immune cells may be engaged in mediating immune responses upon POLθ inhibition, as the proportions of CD11c + CD11b − dendritic cells (DCs) and CD11b + CD11c − macrophages were also increased (Fig. 2g, h ; Supplementary Figs. 2a , 3a, b ). To evaluate the importance of a T-cell-mediated immune response for the antitumor efficacy of NVB, we depleted CD8 + T cells using an anti-CD8 antibody in both syngeneic models of BRCA-deficient cancers and treated with vehicle or NVB. Antibody-mediated depletion of CD8 + T cells decreased the tumor growth inhibition mediated by NVB (Fig. 2i, j ; Supplementary Fig. 2c–e ). Thus, we conclude that CD8 + T cells are required for NVB-mediated POLθ inhibition to be fully effective in vivo. Fig. 2: Efficacy of POLθ inhibition in HR-deficient cancers requires CD8 + T cells. a , b K14-Cre-Brca1 f/f ;Trp53 f/f TNBC tumors from syngeneic FVB/129P2 mice (VEH, n = 5; NVB, n = 7) ( a ), or Brca2 KO KPC PDAC tumors from syngeneic C57BL/6 mice (VEH, n = 7; NVB, n = 6) ( b ) were subjected to IHC for CD3, CD4, and CD8 expression. Left: Representative IHC images at 40x magnification, scale bars, 100 μM. Right: Quantification of IHC using Aperio algorithms. Data, mean +/−SEM, unpaired two-tailed t- tests. c , d K14-Cre-Brca1 f/f ;Trp53 f/f tumors TNBC (VEH, n = 7; NVB, n = 6) ( c ), or Brca2 KO KPC PDAC tumors (VEH, n = 10; NVB, n = 9) ( d ) were harvested 5 days after treatment and analyzed by flow cytometry. Scatter plots show significant increases in CD45 + , CD3 + , CD8 + , and Granzyme B + cells in NVB-treated animals. Error bars, SEM. Statistical analyses were performed using unpaired two-tailed t- tests. e , f TNBC tumors (VEH, n = 7; NVB, n = 6) ( e ) or PDAC tumors (VEH, n = 10; NVB, n = 9) ( f ) were analyzed by flow cytometry. Scatter plots show CD4 + cells, CD4 + T regulatory (FoxP3 + ) cells. Error bars, SEM. Statistical analyses were performed using unpaired two-tailed t- tests. g , h TNBC tumors (VEH, n = 7; NVB, n = 6) ( g ) or PDAC tumors (VEH, n = 10; NVB, n = 9) ( h ) were analyzed by flow cytometry for macrophages (CD11b + , CD11c-). Error bars, SEM. Statistical analyses were performed using unpaired two-tailed t- tests. i K14-Cre-Brca1 f/f ;Trp53 f/f GEMM tumor-bearing syngeneic FVB/129P2 mice were treated with vehicle ( n = 6) or NVB (75 mg/kg twice daily; n = 8), along with isotype control ( n = 6) or an anti-CD8 antibody (200 µg twice weekly; n = 8) for 28 days. Graph shows the serial fold-change in tumor volume. Data, mean +/−SEM, one-way ANOVA analysis. j Brca2 KO KPC PDAC tumor-bearing syngeneic C57BL/6 mice were treated with vehicle ( n = 9) or NVB (75 mg/kg twice daily; n = 10), along with isotype control ( n = 9) or an anti-CD8 antibody (200 µg twice weekly; n = 10) for 28 days. Graph shows the serial fold-change in tumor volume. Data, mean +/−SEM, one-way ANOVA analysis. Full size image POLθ inhibition activates the cGAS/STING pathway in HR-deficient cancers Mammalian Polq was first identified in a mutagenesis screen for chromosome instability mutants using a flow cytometric peripheral blood micronucleus assay [16] . Micronuclei are a known source of immunostimulatory cytosolic DNA that activates the cGAS/STING pathway, leading to increased expression of type I interferons, as can occur after exposure to other DNA repair pathway inhibitors [12] , [13] , [17] , [24] . Accordingly, we sought to determine whether NVB-induced cytotoxic T-cell recruitment and synergy with anti-PD-1 therapy is mediated by the cGAS/STING pathway, as PD-L1 is an interferon response gene [25] , [26] . To test this hypothesis, we first examined cGAS/STING pathway activation in the MDA-MB-436 and CAPAN-1 isogenic paired cell lines (Fig. 3 ; Supplementary Fig. 4 ). NVB-mediated POLθ inhibition significantly increased cytosolic dsDNA contained in micronuclei in MDA-MB-436 HR-deficient but not BRCA1-reconstituted HR-proficient cells (Fig. 3a ; Supplementary Fig. 4a ). Similar results were observed in CAPAN-1 HR-deficient and BRCA2-reconstituted cells (Fig. 3b ; Supplementary Fig. 4b ). This free DNA was sensed by the cytosolic DNA sensor cyclic GMP-AMP (cGAMP) synthetase (cGAS) in HR-deficient MDA-MB-436 and CAPAN-1 cells but not in their BRCA-reconstituted derivatives (Fig. 3a-d ; Supplementary Fig. 4a, b ) [27] , [28] , [29] , [30] . cGAS mediates the synthesis of cGAMP in response to increased cytosolic dsDNA, and NVB consequently significantly increased cGAMP production only in HR-deficient cells, but not in their HR-proficient counterparts (Fig. 3e, f ). cGAMP binds to and activates stimulator of interferon genes (STING), triggering phosphorylation of TBK1 and ultimately of IRF3. Phosphorylated IRF3 subsequently translocates to the nucleus, where it activates the expression of type I interferon and interferon-responsive genes [23] , [28] , [29] , [30] , [31] . Treatment of HR-deficient cell lines with NVB led to activation of the STING pathway, as evidenced by phosphorylation of STING, STAT1, and TBK1 (Fig. 3g ). Similar results were observed with siRNA-mediated knockdown of POLQ (Fig. 3h ) or with ART558-mediated inhibition of POLθ (Fig. 3i ) in both MDA-MB-436 and CAPAN-1 cells, indicating that the consequences of NVB treatment were unlikely due to off-target effects. To demonstrate that POLθ inhibition also leads to the activation of IRF3 in HR-deficient but not HR-proficient cells, we performed immunofluorescence for phosphorylated IRF3 in MDA-MB-436 or CAPAN-1 cell lines and their BRCA-reconstituted derivatives treated with NVB (Fig. 3j, k ; Supplementary Fig. 4c, d ). Increased phosphorylation and activation of IRF3 correlated with DNA damage accumulation, as evidenced by formation of γH2AX foci upon NVB treatment (Fig. 3l, m ). Fig. 3: POLθ inhibition activates the cGAS/STING pathway in BRCA-deficient cancers. a – d The pair of MDA-MB-436 +/− BRCA1 isogenic cell lines ( a ), or the pair of CAPAN-1 +/− BRCA2 isogenic cell lines ( b ) were treated with vehicle (VEH) or 100 μM NVB for 48 h, fixed and stained with picogreen, and subjected to immunofluorescence (IF) for cGAS. a , b and Supplementary Fig. 3a, b , Representative IF images at 100x magnification, scale bars, 10 μM. c , d Quantification of the number of cGAS-colocalized micronuclei expressed as a percentage of total nuclei ( n = 100 imaged cells / treatment group). Significance of difference determined by one-way ANOVA. e , f Analysis of 2′3′-cGAMP levels by ELISA in the isogenic cell line pair MDA-MD-436 +/− BRCA1 ( e ), and the isogenic cell line pair CAPAN-1 +/− BRCA2 ( f ) treated with VEH or 100 μM NVB for 48 h. Data, mean +/− SD of three independent experiments, one-way ANOVA. g MDA-MD-436 (left) and CAPAN-1 (right) cell lines cell lines were treated with VEH or 100 μM NVB for 48 h and whole-cell lysates were subjected to immunoblotting with representative immunoblot of three independent experiments. h MDA-MD-436 (left) and CAPAN-1 (right) cell lines cell lines were transfected with siRNA targeting POLQ and whole-cell lysates were subjected to immunoblotting with representative immunoblot of three independent experiments. i MDA-MD-436 (left) and CAPAN-1 (right) cell lines were treated with VEH or 1 μM ART558 (ART) for 48 h. Whole-cell lysates were subjected to immunoblotting with representative immunoblot of three independent experiments. j , k Isogenic cell line pairs (MDA-MD-436 +/− BRCA1, j ) and (CAPAN-1 +/− BRCA2, k ) were treated with DMSO or 100 μM NVB for 48 h, and subsequently subjected to immunofluorescence for pIRF3 Ser396 . For representative IF images, see Supplementary Fig. 3c, d . Quantification of each cell line ( n = 100 imaged cells/treatment group), data, mean +/− SD, one-way ANOVA. l , m Representative IF images of respective cell lines, MDA-MD-436 ( l ) or CAPAN-1 ( m ), treated with 100 μM NVB for 48 h and subjected to IF for γH2AX and pIRF3 Ser396 . Full size image Since phosphorylated IRF3 is a transcription factor for type I interferon genes, we predicted that NVB would lead to increased mRNA expression of type I interferon genes [32] . Indeed, NVB treatment of BRCA1-deficient MDA-MB-436 or BRCA2-deficient CAPAN-1 cells significantly increased mRNA expression of a panel of type I interferon genes ( ISG15, IRF7, CCL5, CXCL10, and IFNB1 ) (Fig. 4a, b ). Consistently, siRNA-mediated depletion of POLQ or treatment with ART558 similarly increased type I interferon gene mRNA expression (Fig. 4c–f ; Supplementary Fig. 4e–h ). Fig. 4: POLθ inhibition induces an in vitro pro-inflammatory response in BRCA-deficient cancers. a , b MDA-MD-436 ( a ) cells or CAPAN-1 ( b ) were treated with DMSO or 100 μM NVB for 48 h. RNA was extracted and qPCR performed. ISG15 , IRF7 , CCL5 , CXCL10 , and IFNB1 mRNA levels were normalized to ACTB internal control. Data, mean +/−SD of 3 independent experiments, unpaired two-way t- tests. c , d Indicated cell lines (MDA-MD-436, c ; CAPAN-1, d ) were transfected with siRNA targeting POLQ , and RNA was extracted, and qPCR performed. ISG15 , and CCL5 mRNA levels were normalized to ACTB internal control. Data, mean +/−SD of 3 independent experiments. Statistical analyses were performed using unpaired two-tailed t -tests. e , f Indicated cell lines (MDA-MD-436, e ; CAPAN-1, f ) were treated with 1 μM ART558 (ART) for 48 h, and RNA was extracted, and qPCR performed. ISG15 , and CCL5 mRNA levels were normalized to ACTB internal control. Data, mean +/−SD of 3 independent experiments. Statistical analyses were performed using unpaired two-tailed t -tests. g PARP inhibitor (PARPi) sensitive or resistant MDA-MB-436 cell lines were treated with DMSO or 100 μM NVB for 48 h, and whole-cell lysates were subjected to immunoblotting. POLθ inhibition increased TBK1 phosphorylation and PD-L1 expression in both PARPi sensitive and resistant MDA-MB-436 cells, with representative immunoblot of three independent experiments. h PARPi resistant MDA-MB-436 cell lines were treated with DMSO or 100 μM NVB for 48 h, and RNA was extracted, and qPCR performed for ISG15 and CCL5 , normalized to ACTB internal control. Data, mean +/−SD of three independent experiments, unpaired two-tailed t -tests. Full size image Although BRCA-reconstituted cells no longer have MMEJ dependence or NVB sensitivity, we have previously shown that BRCA-deficient cells exposed to graded concentrations of a PARP inhibitor until acquired resistance emerges retain high levels of POLQ expression and NVB sensitivity [5] . We therefore asked whether NVB-mediated POLθ inhibition would also activate the cGAS/STING pathway in the setting of acquired PARP inhibitor resistance, using MDA-MB-436 rucaparib-resistant (MDA-MB-436-RR) cells that are cross-resistant to other PARP inhibitors and cisplatin [21] . Consistent with the persistent sensitivity of PARP inhibitor-resistant cells to POLθ inhibition, we observed robust activation of the cGAS/STING pathway in response to NVB in the resistant cells (Fig. 4g, h ; Supplementary Fig. 4i ). To determine whether NVB would activate the cGAS/STING pathway in HR-deficient cancers in vivo, we performed flow cytometric analysis of both Brca1-deficient TNBC tumors and Brca2-deficient PDAC tumors from immunocompetent mice treated for 5 days with NVB. Consistent with the in vitro data, POLθ inhibition significantly increased the proportion of pTBK1 + CD45 − (Fig. 5a, b ) and pIRF3 + CD45 − cells (Fig. 5c, d ; Supplementary Fig. 5a–c ). In vivo activation of the cGAS/STING pathway consequently led to increased expression of a panel of type I interferon genes (Fig. 5e, f ). Fig. 5: POLθ inhibition induces an in vivo pro-inflammatory response in BRCA-deficient cancers. a – d TNBC tumors from vehicle- or NVB-treated mice from 1h (VEH, n = 7; NVB, n = 6) were harvested 5 days after treatment and analyzed by flow cytometry for TBK1 and pIRF3 expression ( a , c ). PDAC tumors from vehicle- or NVB-treated mice from 1j (VEH, n = 10; NVB, n = 9) harvested 5 days after treatment and analyzed by flow cytometry for TBK1 and pIRF3 expression ( b , d ). Scatter plots show significant increases in pTBK1 + and pIRF3 + in CD45 - cells from NVB-treated animals. Error bars, SEM. Statistical analyses were performed using unpaired two-tailed t- tests. e , f Whole-tumor qPCR was performed on RNA from TNBC (VEH, n = 9; NVB, n = 9) ( e ) or PDAC (VEH, n = 5; NVB, n = 5) ( f ) tumors. Scatter plots show significant increases in Isg15 , Irf7, Ccl5 , Cxcl10 , and Ifnb1 mRNA levels normalized to ACTB control from NVB-treated animals. Error bars, SEM. Statistical analyses were performed using unpaired two-tailed t- tests. Full size image In summary, we conclude that POLθ inhibition activates the cGAS/STING pathway in HR-deficient cancers, accounting for the increased production of type I interferons and recruitment of CD8 + T cells and underlying the decreased efficacy of NVB when combined with anti-CD8 treatment. POLθ inhibition in HR-deficient tumors activates the cGAS/STING pathway in dendritic cells (DCs) NVB treatment of immunocompetent mice bearing Brca-deficient tumors also resulted in an increased proportion of CD11c + CD11b − DCs in the tumor microenvironment (Supplementary Fig. 2a ). Furthermore, NVB-mediated POLθ inhibition led to increased concentration of a potent DC chemokine, CCL5 [33] , in the media of both MDA-MB-436 or CAPAN-1 cells (Supplementary Fig. 5d, e ). Given that the cGAS/STING pathway can be activated in DCs and that NVB treatment activates this pathway in tumor cells, we asked whether cGAS/STING pathway activation is also increased in response to NVB in DCs. Consequent expression of type I interferons would be expected to facilitate tumor antigen presentation on DCs and help activate DCs [28] . Flow cytometric analysis of the CD11c + CD11b − cells derived from either Brac1-deficent TNBC or Brca2-deficient PDAC tumors demonstrated a significant increase in the proportion expressing pTBK1, pIRF3, and PD-L1 after NVB exposure (Fig. 6a, b ; Supplementary Fig. 5f–h ). Fig. 6: POLθ inhibition in HR-deficient tumors induces the cGAS/STING pathway in dendritic cells. a , b TNBC tumors from 1h (VEH, n = 7; NVB, n = 6) or PDAC tumors from 1j (VEH, n = 10; NVB, n = 9), were harvested 5 days after treatment and analyzed by flow cytometry. Scatter plots demonstrate increases in pTBK1 + , pIRF3 + , and PD-L1 in dendritic cells (DCs). Error bars, SEM. Statistical analyses were performed using unpaired two-tailed t -tests. c Human dendritic cells were treated with 100 μM and 200 μM NVB for 48 h. After 48 h of incubation, DCs were collected and processed for qPCR analysis. qPCR analysis of ISG15 , IRF7 , CCL5 , CXCL10 , and IFNB1 mRNA levels normalized to ACTB control. 10 μM ADU-S100 (labeled as STING) was used as a positive control. Data, mean +/− SD of 3 independent experiments, one-way ANOVA. d Illustration of co-culture system using human dendritic cells and NVB-treated tumor cells. HR-deficient tumor cells were treated with vehicle or 100 μM NVB for 48 h, after which were removed and DCs were co-cultured for 24 h. Floating cells representing DCs were collected and processed for qPCR analysis. Created using Biorender. e , f qPCR analysis of ISG15 , IRF7, CCL5, CXCL10 , and IFNB1 mRNA levels normalized to ACTB control in DCs co-cultured with untreated and NVB-treated MDA-MB-436 cells ( e ), or CAPAN-1 cells ( f ). Data, mean +/− SD of 3 independent experiments, unpaired two-tailed t -tests. Full size image To determine if the activation of the cGAS/STING pathway in DCs is a direct effect of NVB, we treated human DCs with increasing concentrations of NVB ex vivo. As a positive control, DCs were also treated with the STING agonist ADU-S100. Whereas treatment of DCs with ADU-S100 enhanced type I interferon gene expression, there was no change in type I interferon gene expression upon NVB treatment (Fig. 6c ). This result suggests that POLθ inhibition does not directly activate the cGAS/STING pathway in DCs. We therefore performed co-culture experiments with DCs together with vehicle- or NVB-treated BRCA1-deficient MDA-MB-436 cells or BRCA2-deficient CAPAN-1 cells (Fig. 6d ). We observed significant enhancement of type I interferon gene expression in DCs co-cultured with NVB compared to vehicle-treated BRCA1-deficient TNBC cells (Fig. 6e ) or BRCA2-deficient CAPAN-1 cells (Fig. 6f ), likely secondary to the increased 2,3 cGAMP observed upon NVB-mediated POLθ inhibition (Fig. 3e, f ). These results indicate NVB-mediated POLθ inhibition in BRCA-deficient cancer activates the cGAS/STING pathway in dendritic cells in a paracrine fashion. cGAS/STING pathway activation is required for the pro-inflammatory response and PD-L1 upregulation mediated by POLθ inhibition We next sought to directly link the pro-inflammatory response and consequent upregulation of PD-L1 expression observed in NVB-treated BRCA-deficient cancers to cGAS/STING pathway activation. To establish dependence of these events on the cGAS/STING pathway, we depleted STING by siRNA in BRCA1-deficient MDA-MB-436 cells and in BRCA2-deficient CAPAN-1 cells and assayed phosphorylated TBK1 levels by immunoblot in response to NVB. Depletion of STING by siRNA abrogated NVB-mediated phosphorylation of TBK1 in both cell lines (Fig. 7a, b ). We then determined if STING depletion would prevent the enhanced type I interferon gene expression observed upon NVB-mediated POLθ inhibition. As predicted, qPCR demonstrated that the enhanced type I interferon gene expression seen upon NVB treatment was abrogated upon STING depletion (Fig. 7c, d ). To confirm that activation of the cGAS/STING pathway is dependent on POLθ inhibition, we depleted POLQ , STING , or both in MDA-MB-436 or CAPAN-1 cells. As expected, POLQ depletion was accompanied by STING pathway activation, evidenced by TBK1 phosphorylation. However, combined deletion of POLQ and STING abrogated TBK1 phosphorylation (Fig. 7e, f ). Additionally, whereas POLQ depletion alone resulted in upregulation of PD-L1 expression, this was also abrogated by combined POLQ and STING depletion (Fig. 7e, f ). These results reflect the ability of type I interferons to upregulate PD-L1 expression [25] . Taken together, these data are consistent with reduced POLθ activity leading to cGAS/STING pathway activation that is required for PD-L1 upregulation. Fig. 7: cGAS/STING pathway activation is required for POLθ inhibition-mediated pro-inflammatory response. a , b MDA-MB-436 ( a ) or CAPAN-1 ( b ) cells were depleted of STING by siRNA and then treated with vehicle or 100 μM NVB for 48 h and subjected to immunoblotting. STING depletion as shown by immunoblotting for STING protein levels, abolishes NVB-mediated TBK1 phosphorylation in MDA-MB-436 ( a ), and CAPAN-1 ( b ) cells. c , d MDA-MB-436 or CAPAN-1 cells depleted of STING by siRNA and treated with 100 μM NVB for 48 h were subjected to qPCR. STING depletion abolishes NVB-mediated upregulation of ISG15 and IRF7 mRNA levels normalized to ACTB control in MDA-MB-436 ( c ), and CAPAN-1 ( d ) cells. Data, mean +/− SD of 3 independent experiments, one-way ANOVA. e , f MDA-MD-436 ( e ) or CAPAN-1 ( f ) cells were depleted of STING , POLQ , or the combination by siRNA and subjected to immunoblotting. Combination STING and POLQ siRNA-mediated depletion, as shown by immunoblotting for STING and POLQ protein levels, abolishes TBK1 phosphorylation and increased expression of PD-L1. Representative immunoblot of three independent experiments. Full size image To determine if STING pathway activation is required for NVB-mediated antitumor efficacy in vivo, we generated Sting KO cells using CRISPR/Cas9 in KPC Brca2 KO cells (Fig. 8a ). KPC Brca2 KO cells were employed since NVB-mediated POLθ inhibition did not activate the cGAS/STING pathway in KPC cells (Supplementary Fig. 6 ). We next confirmed that these KPC Brca2 Sting double knockout (DKO) cells did not activate a pro-inflammatory response upon NVB treatment compared to KPC Brca2 KO cells. As expected, CRISPR/Cas9-mediated depletion of Sting abrogated both NVB-mediated phosphorylation of TBK1 and enhanced type I interferon gene expression (Fig. 8b ; Supplementary Fig. 7a ). Consequently, CRISPR/Cas9-mediated depletion of Sting abrogated NVB-mediated upregulation of PD-L1 expression (Fig. 8c ). To directly assess the requirement of cGAS/STING pathway activation in the antitumor efficacy of NVB, we implanted KPC Brca2 KO or KPC Brca2 Sting DKO cells into syngeneic mice and treated with NVB. Consistent with our previous results, NVB treatment significantly increased the mRNA expression of pro-inflammatory type I interferons in KPC Brca2 KO tumors (Fig. 8d , Supplementary Fig. 7b ) and the proportion of infiltrating T cells (Fig. 8e, f ), an effect that was lost in the Brca2 Sting DKO PDAC tumors (Fig. 8d–f ; Supplementary Fig. 7b ). Notably, PD-L1 expression was also significantly decreased in the Brca2 Sting DKO PDAC tumors despite NVB-mediated POLθ inhibition, consistent with our in vitro data, supporting a direct role for POLθ inhibitor-mediated cGAS/STING activation in the upregulation of PD-L1 (Fig. 8e, f ). As previously observed, tumor volume was significantly reduced in response to NVB in mice bearing KPC Brca2 KO cells; however, the antitumor efficacy of NVB was significantly impaired in STING-depleted tumors (Fig. 8g ; Supplementary Fig. 7c ). These results demonstrate that NVB-mediated POLθ inhibition activates the cGAS/STING pathway leading to a pro-inflammatory response that is required for antitumor efficacy in vivo. Fig. 8: cGAS/STING pathway activation is required for POLθ inhibition-mediated antitumor efficacy and immune checkpoint activation. a Immunoblot analysis of STING protein expression in Sting CRISPR knockout KPC Brca2 KO cells. Tubulin serves as an internal loading control. Representative immunoblot of three independent experiments. b Immunoblot analysis of TBK1 phosphorylation in KPC Brca2 KO cells and KPC Brca2 Sting DKO cells upon 100 μM NVB treatment for 48 h. Sting depletion abolishes NVB-mediated Tbk1 phosphorylation. Representative immunoblot of three independent experiments. c Immunoblot analysis of PD-L1 expression in KPC Brca2 KO cells and KPC Brca2 Sting DKO cells upon 100 μM NVB treatment for 48 h. Sting depletion abolishes NVB-mediated PD-L1 upregulation. Representative immunoblot of three independent experiments. d PDAC tumors ( Brca2 KO, or Brca2 Sting DKO from vehicle- or twice daily 75 mg/kg NVB-treated mice ( n = 5 per treatment group) were harvested 5 days after treatment and analyzed by whole-tumor qPCR. Scatter plots show significant increases in Isg15 and Irf7 . mRNA levels normalized to ACTB control from NVB-treated animals harboring Brca2 KO PDAC tumors but not Brca2 Sting DKO PDAC tumors. Error bars, SEM. Statistical analyses were performed using one-way ANOVA. e , f PDAC tumors Brca2 KO (VEH, n = 5; NVB, n = 5), or Brca2 Sting DKO (VEH, n = 5; NVB, n = 6) from vehicle- or twice daily 75 mg/kg NVB-treated mice were harvested 5 days after treatment and analyzed by IHC for CD3, CD4, CD8, and PD-L1 expression. Representative IHC images at 40x magnification, scale bars, 100 μM ( e ). Quantification of IHC staining using Aperio algorithms. Data, mean +/− SEM, unpaired two-tailed t- tests ( f ). g KPC Brca2 KO (VEH, n = 10; NVB, n = 10) or KPC Brca2 Sting DKO (VEH, n = 10; NVB, n = 10) cells were transplanted in syngeneic C57/BL6 mice and treated with vehicle (VEH) or NVB. Tumor volumes (mm 3 ) were measured at days 5 and 22. Error bars, SEM. Statistical analysis was performed using unpaired two-way t- tests. Full size image Here we report that POLθ inhibition enhances PD-L1 expression in BRCA1-deficient breast and BRCA2-deficient pancreatic cancer cells but not in BRCA-reconstituted isogenic pairs. Consequentially and significantly, the antitumor activity of POLθ inhibition is augmented by anti-PD-1 immunotherapy in a Brca2-deficient mouse model of PDAC, representing a novel therapeutic strategy to sensitize HR-deficient cancers to immunotherapy. This effect is mediated through recruitment of cytotoxic granzyme B-positive CD8 + T cells, along with paracrine activation of DCs. Depletion of CD8 + T cells decreased the antitumor efficacy of POLθ inhibition. Mechanistically, POLθ inhibition in BRCA-deficient, but not in BRCA-proficient cancer cells, induced significant micronucleation likely related to the recently recognized role of POLθ in DSB repair during mitosis [34] , causing progression through mitosis with residual DSBs, which leads to micronuclei formation [35] . This resulted in intratumoral activation of the cGAS/STING pathway and enhanced expression of type I interferon genes, including PD-L1. Depletion of STING in tumor cells abolished the pro-inflammatory response mediated by POLθ inhibition, prevented recruitment of CD8 + T cells, and abrogated increased PD-L1 expression. Importantly, results were similar with two different POLθ inhibitors, NVB and ART558, indicating that inhibition of either the ATPase domain or the polymerase domain of POLθ can modulate the tumor immune microenvironment. Our findings demonstrate that POLθ inhibition combined with immunotherapy has significant antitumor effects, suggesting that this combination could be clinically valuable in cancers not thought historically responsive to immunotherapy, such as PDAC. 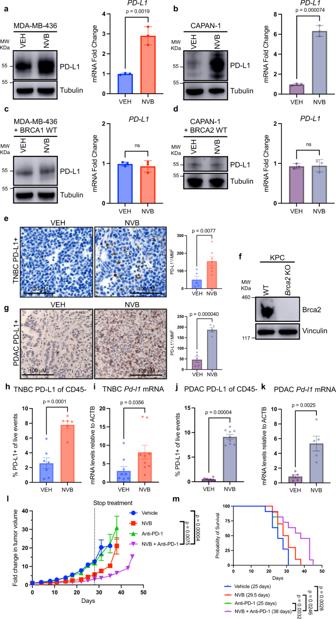Fig. 1: POLθ inhibition induces PD-L1 expression in vitro and in vivo and is enhanced by anti-PD-1 immunotherapy in HR-deficient cancers. a–dBRCA1-mutant MDA-MB-436 TNBC (a) cells, orBRCA2-mutant CAPAN-1 PDAC (b) cells, and their isogenic pairs, BRCA1-expressing MDA-MB-436 (c), or BRCA2-expressing CAPAN-1 (d), were exposed to 100 μM novobiocin (NVB) for 48 h. Left: Immunoblot for PD-L1 expression. Right: Quantification ofPD-L1mRNA levels by RT-qPCR. Transcript levels are measured relative toACTBby qPCR. Data, mean +/− SD of three independent experiments, unpaired two-tailedt-test.eTumor chunks derived from theK14-Cre-Brca1f/f;Trp53f/fGEMM were transplanted in syngeneic FVB/129P2 mice treated with vehicle (VEH,n= 5) or NVB (n= 7) at 75 mg/kg via intraperitoneal (IP) injection twice daily, were harvested after 5 days of treatment for PD-L1 expression by IHC. Staining was quantified using Aperio algorithms. (Left: Representative IHC images at 40x magnification, scale bars, 100 μM. Right: Quantification, Data, mean +/− SEM, unpaired two-tailedt-test.fImmunoblot analysis of Brca2 protein expression in CRISPR knockoutKrasLSL-G12D; TP53LoxP; Pdx1-Cre; Rosa26YFP/YFP(KPC) cells. Vinculin serves as an internal loading control. Representative immunoblot of three independent experiments.gBrca2KO KPC cells were injected into the flanks of syngeneic C57BL/6 mice and treated with VEH(n= 5) or NVB (n= 5) at 75 mg/kg via IP injection twice daily. After 5 days of treatment, tumors were harvested and subjected to IHC for PD-L1 expression. Left: Representative IHC images at 40x magnification, scale bars, 100 μM. Right: Quantification, Data, mean +/− SEM, unpaired two-tailedt-test.h,iPD-L1 protein (h) or mRNA (i) expression inK14-Cre-Brca1f/f;Trp53f/fTNBC tumors. VEH,n= 7; NVB,n= 6 in (h); VEH,n= 9; NVB,n= 9 in (i).j,kPD-L1 protein (j) or mRNA (k) expression inBrca2KO KPC PDAC tumors. VEH,n= 10; NVB,n= 9 in (j); VEH,n= 5; NVB,n= 5 ink. Error bars, SEM. Statistical analyses were performed using unpaired two-tailedt-tests.lBrca2KO KPC tumor-bearing syngeneic C57BL/6 mice were treated with VEH (n= 11) or NVB (75 mg/kg IP twice daily,n= 10), along with isotype control (n= 11) or an anti-PD-1 antibody (200 µg twice weekly,n= 11) for 28 days, and serial fold-change in tumor volume was recorded. Data, mean +/− SEM, one-way ANOVA analysis.mKaplan–Meier analysis for time until tumor progression necessitated euthanasia. Median survivals are shown in parentheses for mice from1l. Kaplan–Meier curves were analyzed by the log-rank test. In addition to harboring mutations in BRCA1 or BRCA2 , which is associated with increased POLQ expression (Supplementary Fig 1e, f ) [8] , [11] , HR-deficient TNBC and PDAC are more likely to harbor mutations in TP53 , which leads to even more pronounced expression of POLQ [36] , [37] . Indeed, increased expression of POLQ is a biomarker of NVB sensitivity [5] , [37] . Thus, it would be expected that BRCA- and TP53-deficient cancers would be particularly sensitive to NVB-mediated POLθ inhibition, leading to micronucleation and potential synergy with immunotherapies such as anti-PD-1 blockade. POLθ inhibitors are under active clinical development, and these hypotheses can now be tested in HR repair-deficient patient populations. Preclinically, POLθ inhibitors, such as NVB or ART558, have demonstrated substantial benefits in HR-deficient models of breast and ovarian cancers, secondary to the synthetic lethality induced by combined loss of HR and MMEJ leading to accumulation of single-stranded DNA intermediates and non-functional RAD51 foci [5] , [6] . We have now extended these findings to demonstrate that POLθ inhibition in HR-deficient TNBC and PDAC cancers in vivo display a cell-extrinsic antitumor mechanism involving the activation of local and systemic antitumor immune responses. This mechanism of POLθ inhibitor-mediated antitumor activity is dependent on underlying HR deficiency, activation of the cGAS/STING pathway, and the recruitment of cytotoxic CD8 + T cells. Our results raise several caveats, as well as new avenues of research. First, our findings were dependent on HR deficiency, as POLθ inhibition in HR-proficient TNBC and PDAC cancers did not activate the cGAS/STING pathway. These results are consistent with the lack of cGAS/STING pathway activation seen upon PARP inhibition in HR-proficient breast or ovarian cancers [12] , [13] . Given the synergy observed between POLθ and PARP inhibition by us and others, it would be expected that combined POLθ and PARP inhibition would even more robustly activate the cGAS/STING pathway in HR-deficient cancers. Additionally, since POLθ inhibition can reverse acquired PARP inhibitor resistance, particularly when mediated by DNA end-resection rewiring [5] , [6] , it will be important to determine if POLθ inhibitors can also modulate the immune microenvironment of PARP inhibitor-resistant cancers in vivo. Our in vitro results suggest this will be the case, as NVB was able to induce cGAS/STING activation in BRCA1 -mutant MDA-MB-436 cells with acquired PARP inhibitor resistance. Therefore, in both PARP inhibitor-sensitive and -resistant backgrounds, a PARP inhibitor/POLθ inhibitor/anti-PD-1 antibody triplet may lead to robust and durable antitumor responses. Second, the pro-inflammatory response mediated by POLθ inhibition was dependent on the cGAS/STING pathway. Depletion of STING by siRNA prevented phosphorylation of TBK1 and consequent type I interferon gene expression and prevented increased PD-L1 expression in response to POLθ inhibition or POLQ depletion. Consistent with these effects, intratumoral CRISPR knockout of Sting decreased PD-L1 expression upon NVB treatment of Brca2-deficient PDAC in vivo. Thus, upregulation of PD-L1 expression secondary to POLθ inhibition or depletion likely occurs directly by cGAS/STING activation through the observed upregulation of IFNB1 . Although PD-L1 upregulation has been more strongly linked to type II interferons, it may also be upregulated by a type I response [25] . Similar findings were observed with PARP or CHK1 inhibition [24] , reinforcing the importance of cGAS/STING pathway activation in mediating the response to DNA damage inhibitors [12] , [24] . STING agonists are currently under clinical investigation in combination with chemotherapy or with immunotherapy [34] , raising the question of whether the antitumor efficacy of NVB-mediated POLθ inhibition could be augmented by STING agonism, similar to the improved antitumor response of combined STING agonism and PARP inhibition in Brca1-deficient TNBC [38] . Finally, our work has largely interrogated the T-cell component of the tumor microenvironment in response to POLθ inhibition. Other DNA repair inhibitors, including PARP inhibitors, have been reported to also modulate other immune cell populations, with complex effects on the phenotype of tumor-associated macrophages [39] . In fact, PARP inhibition in Brca1-deficient TNBC resulted in the recruitment of immune-suppressive macrophages [39] , [40] . This avenue of research is especially important given that preliminary data from clinical trials have not yet confirmed that the addition of immunotherapy to PARP inhibition improves antitumor responses compared to PARP inhibitor monotherapy [41] , raising the possibility that depletion or repolarization of macrophages will be necessary to realize the full potential of combined PARP and immune checkpoint blockade. Indeed, we observed increased infiltration of macrophages in response to POLθ inhibition, not only in the same immunocompetent model of Brca1-deficient TNBC, but also in Brca2-deficient PDAC. Further work will be required to assess the phenotype of this macrophage population and whether it is programmed as antitumor or immunosuppressive [42] . Additional studies will be necessary to carefully assess whether other immune cell populations are modulated by POLθ inhibition and whether they are immunostimulatory or suppressive, so that the immune microenvironment can be manipulated to maximize antitumor responses. In summary, POLθ inhibition in HR-deficient TNBC and PDAC mouse models led to cGAS-STING-mediated expression of type I interferons known to be required for optimal immunological control of cancer, thereby resulting in increased immunogenicity of otherwise immunosuppressed tumors such as PDAC [43] . Activation of the cGAS/STING pathway also led to enhanced expression of PD-L1, providing a rationale for investigating the role of immunotherapy in combination with POLθ inhibition. Moreover, our results demonstrating the improved efficacy of the combination of PD-1 blockade with POLθ inhibition provide a strong scientific rationale for combining these modalities in clinical trials. Since POLθ inhibitors are only just entering early phase clinical trials (e.g., NCT04991480 and NCT05687110), it will be important to confirm our preclinical findings of cGAS/STING pathway activation and increased CD8 + T-cell recruitment using paired tumor biopsies to interrogate the immune microenvironment. Such efforts to understand the scope of biological effects mediated by POLθ inhibition will ultimately inform patient stratification, predictive biomarkers, and rational combinatorial strategies. Cell lines Human TNBC BRCA1 -deficient MDA-MB-436 isogenic pairs were grown in RPMI (Gibco) supplemented with 10% FBS and have been previously described [21] . Human MDA-MB-436 rucaparib-resistant (MDA-MB-436-RR) cells that are cross-resistant to other PARP inhibitors and cisplatin were grown in RPMI supplemented with 10% FBS as previously described [21] . Human pancreatic cancer BRCA2 -deficient CAPAN-1 isogenic pairs were a gift from Dr. Christopher Lord and were grown in DMEM (Gibco) supplemented with 20% FBS. The murine pancreatic cancer cell line ( Kras LSL-G12D ; Trp53 LoxP- ; Pdx1-Cre; Rosa26YFP/YFP , referred to as KPC) was derived from late-stage primary tumors from an autochthonous mouse model of Kras and TP53- mutated PDAC, as previously described [23] . These cells were cultured in DMEM (Gibco) supplemented with 10% FBS and were used to generate Brca2 -deficient KPC cells using the CRISPR-based multi-guide Gene Knockout Kit v2 (Synthego). Three guides (AAAGCUCCUCAAACCAAUUG, UUAUACUCAGAUUCCUCCGG, GAAGCAAACUGAUGGUAGGG) targeting murine Brca2 were electroporated. 48 h post-electroporation, genomic DNA was extracted and analyzed by DNA sequencing to confirm the disruption of the functional Brca2 allele and confirmed by Western blot analysis. Similarly, KPC Brca2 cells were used to generate KPC Brca2/Sting DKO cells, also utilizing 3 guides (GCGAGGCUAGGUGAAGUGCU, GAUGAUCCUUUGGGUGGCAA, ACCUGCAUCCAGCCAUCCCA). Human dendritic cells were obtained from Lonza (CC-2701) and cultured in RMPI (Gibco) containing 10% FBS, 800 U/mL GM-CSF (R&D Systems), and 800 U/mL IL-4 (R&D Systems). For co-culture of tumor cells and dendritic cells, 3 × 10 5 tumor cells were cultured in a 6-well plate and treated with DMSO or NVB. After 48 h, media was removed, and tumor cells washed twice with PBS. Media containing 3 × 10 5 human dendritic cells was added and co-cultured for 24 h. Co-cultured cells were harvested for flow cytometry analysis and floating cells and floating cells (representing ~90% dendritic cells) were collected for mRNA analysis. All cell lines were regularly tested for Mycoplasma using MycoAlert Mycoplasma Detection Kit from Lonza and identified by the DFCI Molecular Diagnostics Core Human Cell Line Authentication service at periodic intervals during the course of the study. In vivo experiments All animal experiments were approved by the Institutional Animal Care and Use Committee at the Dana-Farber Cancer Institute (protocol 17-032). Animals were maintained in housing rooms under controlled environmental conditions (temperature: 20+/− 2 °C; humidity: 35+/− 10%; photoperiod: 12 h light/12 h dark; HEPA-filtered air; animals enclosures provided sterile and adequate space with bedding material, food and water, environmental and social enrichment) at the Dana-Farber Cancer Institute Animal Resource Facility. For expansion of the Brca1-deficient TNBC model, tumor pieces generated from K14-Cre-Brca1 f/f ;Trp53 f/f female mice were orthotopically transplanted into the mammary fat pad of 8-week-old first-generation female FVB/129P2 mice that were bred from FVB females (Jackson Laboratories) and 129P2 males (Envigo). For expansion of the Brca2-deficient PDAC model, cultured Brca2 CRISPR-KO KPC or Brca2 Sting CRISPR-DKO cells were harvested and resuspended in DMEM and mixed 1:1 with Matrigel (Corning). A total volume of 0.2 mL containing 2 × 10 6 cells were injected subcutaneously into the flank of female 8-week-old C57BL/6J mice (Jackson Laboratories). For efficacy studies, treatments were started once the tumors were palpable and reached a volume of 50 to 100 mm 3 and continued until tumors either reached 2000 mm 3 in volume or ulcerated more than 10 mm in diameter, at which point mice were euthanized. For flow cytometry studies, mice bearing tumors of ~300 mm 3 in volume were treated with PBS or NVB for 5 days prior to harvesting. These same tumors were also harvested for IHC and for whole-tumor mRNA extraction. PBS-reconstituted NVB was diluted in PBS (Corning) immediately before 0.2 mL intraperitoneal injection and administered at 75 mg/kg twice daily. Anti-CD8 and IgG2b isotype control antibodies (Bio X Cell; #BE0117 and BE0090) were dissolved in PBS (Corning) and administered intraperitoneally at 0.2 mg/dose in a volume of 0.2 mL, respectively, twice per week. Anti-PD-1 and IgG2a isotype control antibodies (Bio X Cell; #BP0273 and BP0089) were dissolved in PBS (Corning) and administered intraperitoneally at 0.2 mg/dose in a volume of 0.2 mL, respectively, twice per week. Tumors were measured every 3 to 4 days using electronic calipers, and tumor volumes were calculated as follows: V = ( W (2) × L )/2. Compounds NVB (Selleckchem, NSC 2382) was reconstituted in DMSO at the indicated concentrations for in vitro studies and in PBS at 75 mg/kg for in vivo studies. ART558 (MedChemExpress, HY-141520) was reconstituted in DMSO and used at a concentration of 1 μM in vitro. ADU-S100 (MedChemExpress, MIW815) was reconstituted in DMSO and used at a concentration of 10 μM in vitro. Flow cytometry Following 5 days of treatment with vehicle (PBS) or NVB at 75 mg/kg, mice were sacrificed, and cardiac perfusion was performed. Tumors were excised, finely minced before being blended with the gentleMACS Dissociator (Miltenyi Biotec) and digested with the MACS Miltenyi Tumor Dissociation Kit (Miltenyi Biotec #130-096-730) according to the manufacturer’s instructions. Dissociated tumor cells were washed with RPMI (Gibco) and lysed with RBC Lysis Solution (Qiagen). Cells were resuspended in fluorescence-activated cell sorting (FACS) buffer composed of PBS, 0.5% BSA, and 2 mM EDTA. Cells were then incubated with the Zombie Aqua Fixable Viability Kit in combination with anti-mouse CD16/CD32 Fcγ receptor II/III blocking antibody (Affymetrix #14-0161-85) for 20 min at RT, prior to incubation with primary antibodies as indicated in Supplementary Table 1 for 1 h at 4 °C. Fixation and permeabilization was performed using the FoxP3/Transcription Factor Staining Buffer Set (Affymetrix #00-5523-00), according to the manufacturer’s guidelines, and incubated with antibodies for intracellular antigens as indicated in Supplementary Table 1 overnight at 4 °C. The following day, cells were washed, resuspended in PBS, and analyzed using a BD LSR Fortessa flow cytometer. Compensation was performed manually using single color and isotype controls as previously described [12] . All-stain, unstained and isotype controls were used to define signal thresholds. Analysis was performed using FlowJo V10 and GraphPad Prism V9. Gating strategies are provided in Supplementary Fig. 1 and Supplementary Fig. 5 . Immunohistochemistry (IHC) IHC was performed on extracted tumors fixed overnight using 10% formalin solution using a Leica Bond automated staining platform. Fixed tumors were paraffin embedded by the Specialized Histopathology Core at the Brigham and Women’s Hospital (BWH). Thin section slides were produced and washed with Histo-Clear II (National Diagnostics HS-202) twice, 100% ethanol twice, and rehydrated with washes of 90%, 80%, 70%, and 50% ethanol. Antigens were unmasked by heating sections to 100 °C with ER2 buffer for 20 min. Once cooled, sections were washed sequentially with Peroxide Block for 5 min and three times with Bond Wash buffer. Sections were then stained in blocking buffer containing primary antibody (Supplementary Table 1 ) for 1 h at RT. Sections were then washed three times with 1X PBS and incubated with linker antibody at 2.5 μg/mL for 8 min followed by two washes with Bond Wash buffer and incubated with polymer for 8 min. Sections were then washed five times with Bond Wash buffer, incubated with Mixed DAB Refine for 10 min, washed three times with deionized water, and incubated with Hematoxylin for 10 min, followed by thrice washing with Bond Wash buffer. Stained slides were scanned on an Olympus BX41 microscope equipped with a digital camera at 40X magnification into the Aperio image analysis platform for algorithmic image analysis. Immunofluorescence Cells were seeded on coverslips and treated as indicated. Cells were washed once with PBS and then fixed using 4% paraformaldehyde for 10 min at RT. Fixed cells were washed twice with PBS before permeabilization with 0.5% Triton X-100 in PBS (PBST) for 5 min at 4 °C. All subsequent wash steps were with PBST. Following permeabilization, cells were washed twice, and then incubated with the appropriate primary antibody (Supplementary Table 1 ) for 1 h at 37 °C. Following primary incubation, cells were washed three times, then incubated with the appropriate secondary antibody (Supplementary Table 1 ) for 1 h at 37 °C. Following secondary incubation, coverslips were washed four times and then mounted on glass slides using mounting media containing DAPI (Vectashield). Cells were imaged using a Zeiss AxioObserver microscope and quantified using Image J (NIH). Immunoblotting Cells were lysed in NETN buffer (10 mM TrisCl, pH 7.4, 1 mM EDTA, 0.05% Nonidet P-40, and protease inhibitors) containing 150 mM NaCl for 15 min on ice. Protein was quantified using Protein Assay Dye Reagent (Bio-Rad) and equal amounts were resolved on Nu-Page Bis-Tris (Invitrogen) polyacrylamide gels using MES buffer and transferred to nitrocellulose membranes using Tris-Glycine wet transfer. Membranes were blocked with 5% milk in TBST for 1 h at RT, and then probed with primary antibodies (Supplementary Table 1 ) for 1 h at RT. Appropriate enhanced chemiluminescence secondary antibodies (Supplementary Table 1 ), were then applied for 1 h at RT. Immunodetection was performed using Western Lightning (Perkin Elmer) and imaged on an AI600 Chemiluminescent Imager (Amersham). cGAMP, CCL5 ELISA Cell lysates from vehicle (DMSO) and NVB-treated cells were prepared in mammalian protein extraction reagent (Thermofisher). Protein concentration of the lysates was determined, and 25 mg of lysate was used to assess either cGAMP or CCL5 levels using an enzyme-linked immunosorbent assay (ELISA) according to the manufacturer’s protocol (Cayman Chemical, #501700, and R&D Systems, DNR00B, respectively). Quantitative PCR (qPCR) RNA was isolated using the Qiagen RNeasy kit (#74104) per the manufacturer’s protocol. RNA yield was quantified by Nanodrop and reverse transcribed using the SuperScript IV First-Strand Synthesis System (Invitrogen) per the manufacturer’s protocol. qPCR was performed using PrimeTime qPCR Probe Assays (IDTDNA) in QuantStudio 7 Real-Time PCR System (Thermofisher) and the delta-delta Ct method (2 –∆∆Ct) was used to calculate in Microsoft Excel the relative fold gene expression of samples using ACTB as a control. 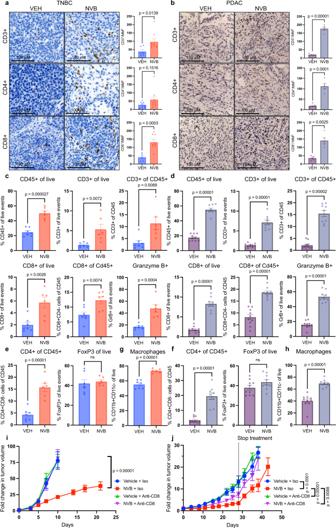Fig. 2: Efficacy of POLθ inhibition in HR-deficient cancers requires CD8+T cells. a,bK14-Cre-Brca1f/f;Trp53f/fTNBC tumors from syngeneic FVB/129P2 mice (VEH,n= 5; NVB,n= 7) (a), orBrca2KO KPC PDAC tumors from syngeneic C57BL/6 mice (VEH,n= 7; NVB,n= 6) (b) were subjected to IHC for CD3, CD4, and CD8 expression. Left: Representative IHC images at 40x magnification, scale bars, 100 μM. Right: Quantification of IHC using Aperio algorithms. Data, mean +/−SEM, unpaired two-tailedt-tests.c,dK14-Cre-Brca1f/f;Trp53f/ftumors TNBC (VEH,n= 7; NVB,n= 6) (c), orBrca2KO KPC PDAC tumors (VEH,n= 10; NVB,n= 9) (d) were harvested 5 days after treatment and analyzed by flow cytometry. Scatter plots show significant increases in CD45+, CD3+, CD8+, and Granzyme B+cells in NVB-treated animals. Error bars, SEM. Statistical analyses were performed using unpaired two-tailedt-tests.e,fTNBC tumors (VEH,n= 7; NVB,n= 6) (e) or PDAC tumors (VEH,n= 10; NVB,n= 9) (f) were analyzed by flow cytometry. Scatter plots show CD4+cells, CD4+T regulatory (FoxP3+) cells. Error bars, SEM. Statistical analyses were performed using unpaired two-tailedt-tests.g,hTNBC tumors (VEH,n= 7; NVB,n= 6) (g) or PDAC tumors (VEH,n= 10; NVB,n= 9) (h) were analyzed by flow cytometry for macrophages (CD11b + , CD11c-). Error bars, SEM. Statistical analyses were performed using unpaired two-tailedt-tests.iK14-Cre-Brca1f/f;Trp53f/fGEMM tumor-bearing syngeneic FVB/129P2 mice were treated with vehicle (n= 6) or NVB (75 mg/kg twice daily;n= 8), along with isotype control (n= 6) or an anti-CD8 antibody (200 µg twice weekly;n= 8) for 28 days. Graph shows the serial fold-change in tumor volume. Data, mean +/−SEM, one-way ANOVA analysis.jBrca2KO KPC PDAC tumor-bearing syngeneic C57BL/6 mice were treated with vehicle (n= 9) or NVB (75 mg/kg twice daily;n= 10), along with isotype control (n= 9) or an anti-CD8 antibody (200 µg twice weekly;n= 10) for 28 days. Graph shows the serial fold-change in tumor volume. Data, mean +/−SEM, one-way ANOVA analysis. Primer sequences are tabulated in Supplementary Table 2 . siRNA transfection For siRNA transfection, cells were seeded at 1 × 10 5 cells/mL into 6-well plates one day prior to planned transfection. Specific siRNA duplexes targeting POLQ (Qiagen SI00090062) or STING (Santa Cruz sc-92042) were transfected using Lipofectamine RNAiMAX Reagent (Life Technologies) according to the manufacturer’s protocol. 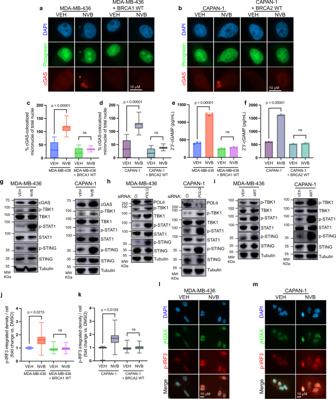Fig. 3: POLθ inhibition activates the cGAS/STING pathway in BRCA-deficient cancers. a–dThe pair of MDA-MB-436 +/− BRCA1 isogenic cell lines (a), or the pair of CAPAN-1 +/− BRCA2 isogenic cell lines (b) were treated with vehicle (VEH) or 100 μM NVB for 48 h, fixed and stained with picogreen, and subjected to immunofluorescence (IF) for cGAS.a,band Supplementary Fig.3a, b, Representative IF images at 100x magnification, scale bars, 10 μM.c,dQuantification of the number of cGAS-colocalized micronuclei expressed as a percentage of total nuclei (n= 100 imaged cells / treatment group). Significance of difference determined by one-way ANOVA.e,fAnalysis of 2′3′-cGAMP levels by ELISA in the isogenic cell line pair MDA-MD-436 +/− BRCA1 (e), and the isogenic cell line pair CAPAN-1 +/− BRCA2 (f) treated with VEH or 100 μM NVB for 48 h. Data, mean +/− SD of three independent experiments, one-way ANOVA.gMDA-MD-436 (left) and CAPAN-1 (right) cell lines cell lines were treated with VEH or 100 μM NVB for 48 h and whole-cell lysates were subjected to immunoblotting with representative immunoblot of three independent experiments.hMDA-MD-436 (left) and CAPAN-1 (right) cell lines cell lines were transfected with siRNA targetingPOLQand whole-cell lysates were subjected to immunoblotting with representative immunoblot of three independent experiments.iMDA-MD-436 (left) and CAPAN-1 (right) cell lines were treated with VEH or 1 μM ART558 (ART) for 48 h. Whole-cell lysates were subjected to immunoblotting with representative immunoblot of three independent experiments.j,kIsogenic cell line pairs (MDA-MD-436 +/− BRCA1,j) and (CAPAN-1 +/− BRCA2,k) were treated with DMSO or 100 μM NVB for 48 h, and subsequently subjected to immunofluorescence for pIRF3Ser396. For representative IF images, see Supplementary Fig.3c, d. Quantification of each cell line (n= 100 imaged cells/treatment group), data, mean +/− SD, one-way ANOVA.l,mRepresentative IF images of respective cell lines, MDA-MD-436 (l) or CAPAN-1 (m), treated with 100 μM NVB for 48 h and subjected to IF for γH2AX and pIRF3Ser396. Statistical analyses Statistical analyses were performed using GraphPad Prism V9 software. All data are represented as mean ± SEM (in vivo) or ±SD (in vitro) calculated unless indicated otherwise. Significance was tested using Student’s t -test for comparison of two sets of measurements, or one-way ANOVA with Tukey post hoc test if all sets analyzed or Sidak post hoc if pairs of sets analyzed, for comparison of three or more sets, unless indicated otherwise. 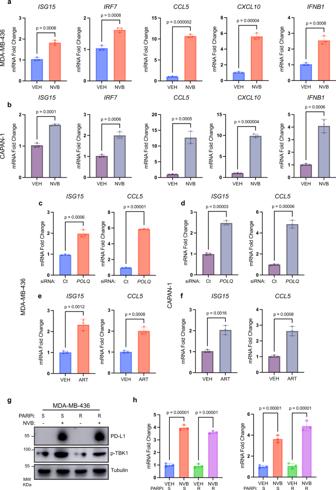Fig. 4: POLθ inhibition induces an in vitro pro-inflammatory response in BRCA-deficient cancers. a,bMDA-MD-436 (a) cells or CAPAN-1 (b) were treated with DMSO or 100 μM NVB for 48 h. RNA was extracted and qPCR performed.ISG15,IRF7,CCL5,CXCL10, andIFNB1mRNA levels were normalized toACTBinternal control. Data, mean +/−SD of 3 independent experiments, unpaired two-wayt-tests.c,dIndicated cell lines (MDA-MD-436,c; CAPAN-1,d) were transfected with siRNA targetingPOLQ, and RNA was extracted, and qPCR performed.ISG15, andCCL5mRNA levels were normalized toACTBinternal control. Data, mean +/−SD of 3 independent experiments. Statistical analyses were performed using unpaired two-tailedt-tests.e,fIndicated cell lines (MDA-MD-436,e; CAPAN-1,f) were treated with 1 μM ART558 (ART) for 48 h, and RNA was extracted, and qPCR performed.ISG15, andCCL5mRNA levels were normalized toACTBinternal control. Data, mean +/−SD of 3 independent experiments. Statistical analyses were performed using unpaired two-tailedt-tests.gPARP inhibitor (PARPi) sensitive or resistant MDA-MB-436 cell lines were treated with DMSO or 100 μM NVB for 48 h, and whole-cell lysates were subjected to immunoblotting. POLθ inhibition increased TBK1 phosphorylation and PD-L1 expression in both PARPi sensitive and resistant MDA-MB-436 cells, with representative immunoblot of three independent experiments.hPARPi resistant MDA-MB-436 cell lines were treated with DMSO or 100 μM NVB for 48 h, and RNA was extracted, and qPCR performed forISG15andCCL5, normalized toACTBinternal control. Data, mean +/−SD of three independent experiments, unpaired two-tailedt-tests. 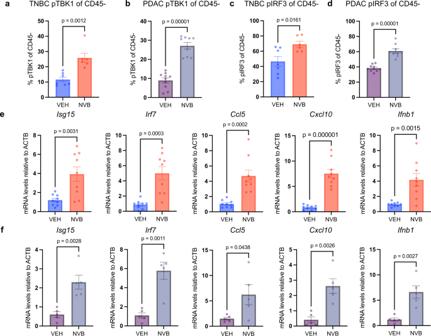Fig. 5: POLθ inhibition induces an in vivo pro-inflammatory response in BRCA-deficient cancers. a–dTNBC tumors from vehicle- or NVB-treated mice from1h(VEH,n= 7; NVB,n= 6) were harvested 5 days after treatment and analyzed by flow cytometry for TBK1 and pIRF3 expression (a,c). PDAC tumors from vehicle- or NVB-treated mice from1j(VEH,n= 10; NVB,n= 9) harvested 5 days after treatment and analyzed by flow cytometry for TBK1 and pIRF3 expression (b,d). Scatter plots show significant increases in pTBK1+and pIRF3+in CD45-cells from NVB-treated animals. Error bars, SEM. Statistical analyses were performed using unpaired two-tailedt-tests.e,fWhole-tumor qPCR was performed on RNA from TNBC (VEH,n= 9; NVB,n= 9) (e) or PDAC (VEH,n= 5; NVB,n= 5) (f) tumors. Scatter plots show significant increases inIsg15,Irf7, Ccl5,Cxcl10, andIfnb1mRNA levels normalized toACTBcontrol from NVB-treated animals. Error bars, SEM. Statistical analyses were performed using unpaired two-tailedt-tests. 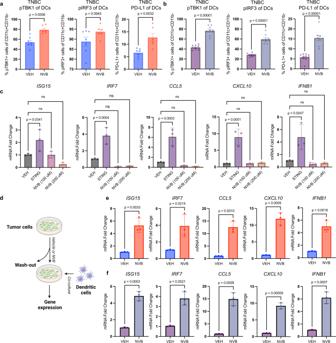Fig. 6: POLθ inhibition in HR-deficient tumors induces the cGAS/STING pathway in dendritic cells. a,bTNBC tumors from1h(VEH,n= 7; NVB,n= 6) or PDAC tumors from1j(VEH,n= 10; NVB,n= 9), were harvested 5 days after treatment and analyzed by flow cytometry. Scatter plots demonstrate increases in pTBK1+, pIRF3+, and PD-L1 in dendritic cells (DCs). Error bars, SEM. Statistical analyses were performed using unpaired two-tailedt-tests.cHuman dendritic cells were treated with 100 μM and 200 μM NVB for 48 h. After 48 h of incubation, DCs were collected and processed for qPCR analysis. qPCR analysis ofISG15,IRF7,CCL5,CXCL10, andIFNB1mRNA levels normalized toACTBcontrol. 10 μM ADU-S100 (labeled as STING) was used as a positive control. Data, mean +/− SD of 3 independent experiments, one-way ANOVA.dIllustration of co-culture system using human dendritic cells and NVB-treated tumor cells. HR-deficient tumor cells were treated with vehicle or 100 μM NVB for 48 h, after which were removed and DCs were co-cultured for 24 h. Floating cells representing DCs were collected and processed for qPCR analysis. Created using Biorender.e,fqPCR analysis ofISG15,IRF7, CCL5, CXCL10, andIFNB1mRNA levels normalized toACTBcontrol in DCs co-cultured with untreated and NVB-treated MDA-MB-436 cells (e), or CAPAN-1 cells (f). Data, mean +/− SD of 3 independent experiments, unpaired two-tailedt-tests. 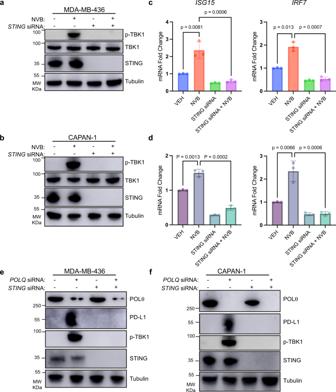Fig. 7: cGAS/STING pathway activation is required for POLθ inhibition-mediated pro-inflammatory response. a,bMDA-MB-436 (a) or CAPAN-1 (b) cells were depleted ofSTINGby siRNA and then treated with vehicle or 100 μM NVB for 48 h and subjected to immunoblotting. STING depletion as shown by immunoblotting for STING protein levels, abolishes NVB-mediated TBK1 phosphorylation in MDA-MB-436 (a), and CAPAN-1 (b) cells.c,dMDA-MB-436 or CAPAN-1 cells depleted ofSTINGby siRNA and treated with 100 μM NVB for 48 h were subjected to qPCR.STINGdepletion abolishes NVB-mediated upregulation ofISG15andIRF7mRNA levels normalized toACTBcontrol in MDA-MB-436 (c), and CAPAN-1 (d) cells. Data, mean +/− SD of 3 independent experiments, one-way ANOVA.e,fMDA-MD-436 (e) or CAPAN-1 (f) cells were depleted ofSTING,POLQ, or the combination by siRNA and subjected to immunoblotting. CombinationSTINGandPOLQsiRNA-mediated depletion, as shown by immunoblotting for STING and POLQ protein levels, abolishes TBK1 phosphorylation and increased expression of PD-L1. Representative immunoblot of three independent experiments. 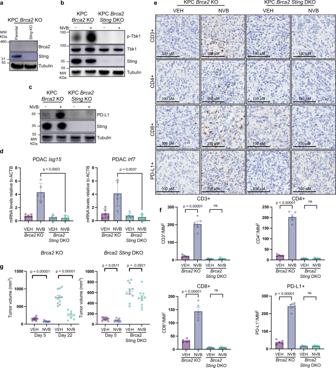Fig. 8: cGAS/STING pathway activation is required for POLθ inhibition-mediated antitumor efficacy and immune checkpoint activation. aImmunoblot analysis of STING protein expression inStingCRISPR knockout KPCBrca2KO cells. Tubulin serves as an internal loading control. Representative immunoblot of three independent experiments.bImmunoblot analysis of TBK1 phosphorylation in KPCBrca2KO cells and KPCBrca2 StingDKO cells upon 100 μM NVB treatment for 48 h. Sting depletion abolishes NVB-mediated Tbk1 phosphorylation. Representative immunoblot of three independent experiments.cImmunoblot analysis of PD-L1 expression in KPCBrca2KO cells and KPCBrca2 StingDKO cells upon 100 μM NVB treatment for 48 h. Sting depletion abolishes NVB-mediated PD-L1 upregulation. Representative immunoblot of three independent experiments.dPDAC tumors (Brca2KO, orBrca2 StingDKO from vehicle- or twice daily 75 mg/kg NVB-treated mice (n= 5 per treatment group) were harvested 5 days after treatment and analyzed by whole-tumor qPCR. Scatter plots show significant increases inIsg15andIrf7. mRNA levels normalized toACTBcontrol from NVB-treated animals harboringBrca2KO PDAC tumors but notBrca2 StingDKO PDAC tumors. Error bars, SEM. Statistical analyses were performed using one-way ANOVA.e,fPDAC tumorsBrca2KO (VEH,n= 5; NVB,n= 5), orBrca2 StingDKO (VEH,n= 5; NVB,n= 6) from vehicle- or twice daily 75 mg/kg NVB-treated mice were harvested 5 days after treatment and analyzed by IHC for CD3, CD4, CD8, and PD-L1 expression. Representative IHC images at 40x magnification, scale bars, 100 μM (e). Quantification of IHC staining using Aperio algorithms. Data, mean +/− SEM, unpaired two-tailedt-tests (f).gKPCBrca2KO (VEH,n= 10; NVB,n= 10) or KPCBrca2 StingDKO (VEH,n= 10; NVB,n= 10) cells were transplanted in syngeneic C57/BL6 mice and treated with vehicle (VEH) or NVB. Tumor volumes (mm3) were measured at days 5 and 22. Error bars, SEM. Statistical analysis was performed using unpaired two-wayt-tests. Reporting summary Further information on research design is available in the Nature Portfolio Reporting Summary linked to this article.